Compact designer TALENs for efficient genome engineering Transcription activator-like effector nucleases are readily targetable ‘molecular scissors’ for genome engineering applications. These artificial nucleases offer high specificity coupled with simplicity in design that results from the ability to serially chain transcription activator-like effector repeat arrays to target individual DNA bases. However, these benefits come at the cost of an appreciably large multimeric protein complex, in which DNA cleavage is governed by the nonspecific FokI nuclease domain. Here we report a significant improvement to the standard transcription activator-like effector nuclease architecture by leveraging the partially specific I-TevI catalytic domain to create a new class of monomeric, DNA-cleaving enzymes. In vivo yeast, plant and mammalian cell assays demonstrate that the half-size, single-polypeptide compact transcription activator-like effector nucleases exhibit overall activity and specificity comparable to currently available designer nucleases. In addition, we harness the catalytic mechanism of I-TevI to generate novel compact transcription activator-like effector nuclease-based nicking enzymes that display a greater than 25-fold increase in relative targeted gene correction efficacy. The application of genome engineering requires the consolidation of many diverse concepts [1] , the most fundamental being the need to specifically and efficiently target a DNA sequence within a complex genome. Reengineering a DNA-binding protein for this purpose has been mainly limited to two semi-modular archetypes [2] , [3] : (i) artificial zinc-finger proteins (ZFP) and (ii) the naturally occurring LAGLIDADG-homing endonucleases (LHE). ZFP targeting relies on the serial chaining of DNA triplet-recognizing zinc-finger motifs and has been successfully used to direct transcription factors [4] , [5] , methylases [6] , [7] , recombinases [8] , [9] and, most commonly, nucleases [10] , [11] (ZFNs). LHEs meanwhile have primarily been used as retargeted nucleases [12] , [13] , [14] , with only a few studies demonstrating their potential as DNA-binding domains per se [15] , [16] . Nevertheless, a common limitation lies in the practical efficiency with which either DNA-binding domain can be produced, with difficulties ranging from time-consuming methods [12] , [13] needed to isolate reengineered variants to deficiencies in the DNA sequence fidelity of the final products [17] , [18] , [19] . A newly characterized class of proteins, derived from transcription activator-like effectors (TALE) identified in plant pathogens of the Xanthomonas genus, is rapidly transforming the state-of-the-art in engineering sequence-specific DNA-binding domains [20] , [21] . TALE binding is driven by a series of 33 to 35 amino-acid-long repeats that differ at essentially two positions, the so-called repeat variable dipeptide (RVD). Each base of one strand in the DNA target is contacted by a single repeat, with predictable specificity resulting from the linear arrangement of RVDs [22] , [23] . Upon elucidation of a DNA recognition ‘code’, a standard cipher was adopted to effectively reengineer TALE DNA-binding scaffold (TDBS) specificity via modular assembly [20] , [21] , [24] . Enhancements to the core TDBS via truncation [24] , [25] , [26] along with the use of additional or alternative RVDs [27] , [28] , [29] have significantly advanced the potential of this programmable DNA-binding domain. TALE engineering has proved surprisingly robust for targeting effector proteins to DNA sequences of interest, including directed transcriptional activators [30] , [31] , [32] and repressors [33] , [34] , as well as TALE-based nucleases [25] , [35] (transcription activator-like effector nucleases (TALENs)). The standard TALEN architecture ( Fig. 1a ) utilizes the requisitely dimeric catalytic domain (CD) of the Type IIS restriction enzyme FokI. TALEN activity thus requires two DNA recognition regions flanking an unspecific central spacer region, with efficiency in DNA cleavage being interdependent with spacer length and TALE scaffold construction [25] , [35] . The highly repetitive nature of the underlying DNA sequence coding for engineered TALEs has made necessary specialized synthesis techniques [24] , [36] , [37] , [38] . Moreover, TALEN halfs are roughly three times larger than canonical designer nucleases, with the overall protein complex generally being >1,800 amino acids. Having to deliver such a large payload, whether as DNA, RNA or protein, necessitates that TALENs offer a substantial improvement over existing technologies. 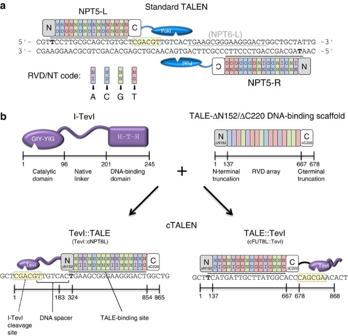Figure 1: Design and creation of cTALENs using the I-TevI CD. (a) Schematic of a standard TALEN architecture overlaid on a sequence fragment of thenptIIgene; RVD designation NPT5. FokI (blue), C-terminal R.FokI DNA-cleavage domain. The default TALE code used for all designs is noted. (b) cTALENs are created by combining the TevI (purple) GIY–YIG CD, fused either N (TevI::TALE) or C terminally (TALE::TevI), with a TDBS. Numbers indicate length in amino acids. TevI cleavage sites are highlighted in the dashed boxes. cNPT6L and cFUT8L, RVD designations for the left TDBS in compact (c) context. Figure 1: Design and creation of cTALENs using the I-TevI CD. ( a ) Schematic of a standard TALEN architecture overlaid on a sequence fragment of the nptII gene; RVD designation NPT5. FokI (blue), C-terminal R.FokI DNA-cleavage domain. The default TALE code used for all designs is noted. ( b ) cTALENs are created by combining the TevI (purple) GIY–YIG CD, fused either N (TevI::TALE) or C terminally (TALE::TevI), with a TDBS. Numbers indicate length in amino acids. TevI cleavage sites are highlighted in the dashed boxes. cNPT6L and cFUT8L, RVD designations for the left TDBS in compact (c) context. Full size image Here, we describe a strategy to overcome these limitations by developing a single-chain TALEN architecture in which a TDBS is fused to the cleavage domain from the I-TevI homing endonuclease [39] . Remarkably, we find that amino-terminal TevI fusions function as natural cleavases, while carboxy-terminal fusions function as natural nickases. These novel compact TALENs (cTALENs) display significant in vivo activity and not only simplify vectorization but straightforwardly reduce production costs and efforts in half for the generation of precision gene-targeting reagents. Designing a single-chain cTALEN In considering design possibilities for the cTALEN ( Table 1 ), we reasoned that a low-affinity cleavage domain that retained some sequence specificity would alleviate accidental off-site cleavage resulting from DNA proximity during target-site scanning by the TALE domain. While it can be envisioned that longer, more-specific TALE domains could themselves eliminate unwanted events by reducing dwell times at non-cognate sites, CD selectivity provides a second level of activity control akin to the FokI dimerization requirement. At the same, a generalized solution was sought for uniform and efficient targeting over a broad range of sequences without having to rely on the presence of an exact sequence match [40] , and also to avoid issues of combined protein engineering ( Table 1 ). For cTALEN fusions, we chose the well-characterized homing endonuclease member of the GIY–YIG protein family, I-TevI [39] , [41] , which exhibits a tripartite protein layout ( Fig. 1b ). The C-terminal domain of I-TevI is responsible for DNA-binding specificity as well as the majority of the protein–DNA interaction affinity. A long, flexible linker tethers and regulates the N-terminal CD that contributes solely to specificity via DNA cleavage selectivity [42] , which has been characterized biochemically in vitro and is defined by the degenerate CN↑NN↓G motif [41] (arrows represent bottom (↑) and top (↓) strand cleavage; natural target sequence: CAACGC). To generate a cTALEN, we opted to replace the I-TevI C-terminal DNA-binding domain by a minimal AvrBs3-derived TALE-ΔN152/ΔC220 scaffold, thereby preserving the natural N to C terminus layout of wild-type I-TevI. This contrasts with standard TALENs having the FokI domain fused at the C terminus ( Fig. 1a ). A final design ( Fig. 1b , left) consisting of the N-terminal 183 residues of wild-type I-TevI fused via a five-residue linker (–QGPSG–) to the N terminus of the TALE scaffold was chosen for further analysis, and is hereafter referred to as TevI::TALE (where ‘TALE’ designates the RVD specificity). Table 1 Design possibilities for cTALEN CDs. Full size table In vivo characterization of the cTALEN As the natural I-TevI linker can act as a distance determinant for DNA cleavage by the CD [42] , we investigated if a similar relationship exists in the context of the artificial TALE fusion. A series of sliding targets ( Fig. 2a ) was generated in which the wild-type I-TevI cleavage sequence is systematically spaced from 0 to 50 base pairs (bp) away from the T 0 of a single AvrBs3 TALE-binding site (TBS), with spacing reported as the distance to the critical terminal G base in the target sequence (CAAC G C). In yeast SSA assays, we observed that TevI::cAvr demonstrates a clear preference for cleavage only of targets having the wild-type sequence, with an effective spacer window of 5 to 15 bp ( Fig. 2a ). Notably, the optimal 10-bp spacer distance, yielding maximal activity equivalent to FokI-based TALENs, is considerably shorter than those of the natural I-TevI [41] (22 bp) and previously engineered TevI-based fusions [15] (~24–28 bps). 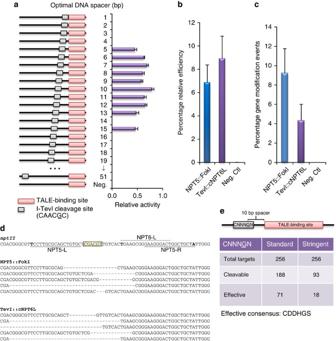Figure 2:In vivocharacterization of TevI-based cTALENs. (a) A series of 52 sliding targets (schematic, left) were generated and tested in a yeast SSA assay (right,n=3) to determine the optimal DNA ‘spacer’ for targeting cleavage. Numbers indicate base count betweenT0of the TBS and the terminal G of the upstream TevI cleavage site. Neg., target lacking a TevI cleavable sequence. (b) TevI-based cTALENs function in tobacco plant protoplasts to induce restoration of a YFP reporter through SSA. TALENs were targeted (n=2) to a sequence fragment of thenptIIgene as noted inFig. 1a. Neg. Ctl, a TevI-based cTALEN targeting a sequence not present in the reporter construct. (c) cTALENs promote targeted gene disruption at endogenous loci. CHO-K1 cells harbouring an integrated neomycin resistance gene were assayed (n=4) with a TALEN or cTALEN targeting the NPT5 or cNPT6L, respectively, overlapping regions. Neg. Ctl as in (b). Gene modification events determined by amplicon sequencing of the target site. (d) Representative mutated alleles detected in amplicon sequencing of cells from (c). Top, referencenptIIgene sequence. Binding sites for the NPT5 TALEN are underlined. The NPT6 cTALEN-binding site is indicated above the sequence, with the upstream TevI cleavage site highlighted. Dashes in the sequence represent deleted bases. (e) Summary of the TevI-based cTALEN specificity profile. ‘CNNNGN’ target sequences, where N represents any base, were generated at a fixed distance from the TBS and evaluated in a yeast SSA assay (n=3) under standard (37 °C) or stringent (30 °C) conditions. Cleavable, targets with an assay value >0. Effective, targets with an assay value >65% of maximal for the condition tested. Data (a–c) are shown as the mean+s.e.m. Neg., negative. Figure 2: In vivo characterization of TevI-based cTALENs. ( a ) A series of 52 sliding targets (schematic, left) were generated and tested in a yeast SSA assay (right, n =3) to determine the optimal DNA ‘spacer’ for targeting cleavage. Numbers indicate base count between T 0 of the TBS and the terminal G of the upstream TevI cleavage site. Neg., target lacking a TevI cleavable sequence. ( b ) TevI-based cTALENs function in tobacco plant protoplasts to induce restoration of a YFP reporter through SSA. TALENs were targeted ( n =2) to a sequence fragment of the nptII gene as noted in Fig. 1a . Neg. Ctl, a TevI-based cTALEN targeting a sequence not present in the reporter construct. ( c ) cTALENs promote targeted gene disruption at endogenous loci. CHO-K1 cells harbouring an integrated neomycin resistance gene were assayed ( n =4) with a TALEN or cTALEN targeting the NPT5 or cNPT6L, respectively, overlapping regions. Neg. Ctl as in ( b ). Gene modification events determined by amplicon sequencing of the target site. ( d ) Representative mutated alleles detected in amplicon sequencing of cells from ( c ). Top, reference nptII gene sequence. Binding sites for the NPT5 TALEN are underlined. The NPT6 cTALEN-binding site is indicated above the sequence, with the upstream TevI cleavage site highlighted. Dashes in the sequence represent deleted bases. ( e ) Summary of the TevI-based cTALEN specificity profile. ‘CNNNGN’ target sequences, where N represents any base, were generated at a fixed distance from the TBS and evaluated in a yeast SSA assay ( n =3) under standard (37 °C) or stringent (30 °C) conditions. Cleavable, targets with an assay value >0. Effective, targets with an assay value >65% of maximal for the condition tested. Data ( a – c ) are shown as the mean+s.e.m. Neg., negative. Full size image We next validated the design for use in plant applications with SSA assays in tobacco protoplasts. A TALEN target site (TTS) was selected in the neomycin phosphotransferase II ( nptII ) gene and a standard FokI-based TALEN (NPT5) was synthesized as control ( Fig. 1a ). An overlapping binding site (NPT6-L) was identified within this target with a requisite CNNNG motif (CGACGT) located 7 bp away to allow for consistent validation of binding and cleavage events within a single TTS. The TevI cTALEN design demonstrated an activity on par with the FokI TALEN (NPT5::FokI, 6.9%; TevI::cNPT6L, 8.9%), with controls confirming that detectable events resulted from targeted gene repair ( Fig. 2b ). To test the cTALEN in mammalian cells, we directly assayed for targeted gene disruption (indels) in a CHO-K1 line containing a single integrated nptII sequence. Amplicon sequencing of genomic DNA showed that the TevI::cNPT6L cTALEN is active (4.3%), being only moderately (~2-fold) less efficient than the NPT5::FokI TALEN counterpart (9.2%) ( Fig. 2c ). Examining the location of the mutagenic events revealed a pattern that follows the overlying protein–DNA interaction for each nuclease ( Fig. 2d ). To better understand the variation in efficacy, we evaluated whether activity differences could be attributed to toxicity or the sequence of the targeted CNNNG motif within the NPT5 TTS. Whereas survival assays in CHO-K1 cells demonstrate no apparent toxicity ( Supplementary Fig. S1 ), benchmarking of the TevI::cNPT6L cTALEN against the NPT5 target in both yeast and CHO-K1 SSA assays revealed a 2- to 3-fold reduction in relative activity compared with a standard TALEN ( Supplementary Fig. S2a,b ). To address how variations in the CNNNG motif can modulate cTALEN activity, a complete series of CNNNGN (N=A, C, G or T) targets was generated, keeping fixed the two key bases thought to most influence activity [41] . Interestingly, whereas in vitro studies of wild-type I-TevI imply that the CD can be indiscriminate [41] , [42] , the cTALEN in vivo data reveal a defined target-site selectivity ( Supplementary Table S1 ). Only 27% of the targets assayed in vivo can be considered effective (as defined by an assay value >65% of maximal) under standard conditions, with 7% cleaved using stringent conditions ( Fig. 2e ). These results indicate that if appropriate CNNNGN targets are chosen, the cTALEN architecture allows for generating reagents as active as FokI-based TALENs, although for less-demanding applications suboptimal CNNNGN motifs may also be used. A working consensus sequence, CDDHGS (D=A, G or T; H=A, C or T; S=C or G), was derived from base rankings at each position but owing to exception complexity only contains 70% effective targets ( Supplementary Table S1 ). Thus, although the cTALEN is active on all targets covered by the consensus sequence, many additional and indeed preferential target sequences exist (for example, the CAGCGT and CAGCGA sequences found in the cNPT6L and cFUT8L targets, respectively). Such a lack of coherence denotes the need for empirically guided target-site selection and may signify an alteration of the TevI catalytic mechanism that is construct dependent. Importantly, these results contrast with recently described TevI-derived nucleases having apparent equivalence in cleavage for all CNNNG motif targets [15] , differences that may reflect alternate constraints imposed by the DNA-binding domain fusion partners utilized. Generation of a cTALEN nickase Wild-type I-TevI functions as a monomer and relies on complex linker interactions to create a DNA double-strand break via a concerted nicking mechanism [39] , [42] . To determine if second-strand cleavage could be uncoupled by disrupting the linker context, we created an inverted C-terminal fusion scaffold termed TALE::TevI ( Fig. 1b , right). In this configuration, although the TevI linker is retained at the C terminus, it can no longer coordinate CD placement relative to the DNA-binding domain. In yeast SSA assays, detectable TALE::TevI activity on single-site targets was highly reduced ( Supplementary Fig. S3a ), yet could be rescued by pairing two molecules in a ‘standard’ TALEN configuration ( Supplementary Fig. S3a,b ). Despite the unnatural fusion layout, TALE::TevI retained cleavage-site selectivity ( Fig. 3a ). These data suggested that perhaps two properly placed nicks were creating the double-strand break. To decipher the TALE::TevI mechanism, we constructed a series of ‘dual-nick’ targets ( Fig. 3b , schematic), hypothesizing that if the TevI domain was always positioned to properly effect the first-strand cleavage, proximity between nicks would govern signal detection. A loss of relative activity was indeed observed as the distance between nicks increased beyond 18 bp ( Fig. 3b ). To confirm that the alternate activity of TALE::TevI was a property of the TevI domain per se , we created a corresponding inverted FokI-based TALEN ( Supplementary Fig. S4a ), which exhibited the expected activity profile similar to a standard TALEN ( Supplementary Fig. S4b ). Taken together, these results demonstrate that differential fusions to a TALE scaffold can be used to regulate the TevI catalytic mechanism, affecting only second-strand cleavage while preserving DNA selectivity. 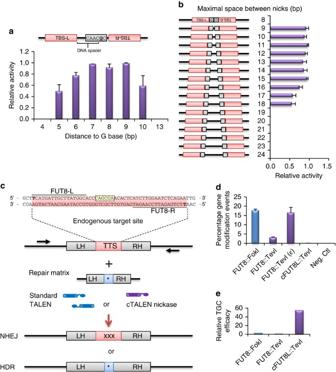Figure 3: Harnessing the TevI domain to create a cTALEN nickase. (a) Optimizing target-site position within the DNA spacer. A series of asymmetric targets (schematic, top) were generated that contain a sliding CAACGC target sequence within a fixed 15-bp DNA spacer region. Relative activity is based on a yeast SSA assay (n=3). TBS-L and TBS-R, TBS for the left and right monomers, respectively. (b) cTALEN nickase activity as a function of DNA spacer. A series of asymmetric targets (schematic, left) were created containing two TBS (TBS-L and TBS-R), each with a flanking TevI target site (C and C′), juxtaposed with the 3′ ends proximal (tail-to-tail) and separated by spacer DNA ranging from 8 to 24 bp between distal nicking sites. Assays (n=3) performed as in (a). (c) Overview of thein vivogene modification assay used for characterizing activity. The repair matrix consists of two homologous regions (LH, left homology; RH, right homology) flanking a 29 bp insert (*). Targeted cleavage stimulates DNA repair either through NHEJ or HDR with the provided matrix, resulting in alternative disruptions (xxx versus *, respectively) of the TTS region. Events are detected via amplicon sequencing using outside primers flanking the homology arms. (d) TevI-based TALENs promote targeted gene disruption at endogenous loci. TALENs targeting the alpha1-6-fucosyltransferase (RVD designation FUT8) gene in CHO-K1 cells were assayed (n=3) as outlined (c) in the absence of a repair matrix. cFUT8L, RVD designation for left TDBS in a cTALEN context. (ε), enhancer reagent TREX2. Neg. Ctl, transfection with empty vector. (e) cTALEN nickases promote TGC. TGC efficacy, calculated as the ratio of HDR:NHEJ events, for assays in CHO-K1 cells as outlined (c) in the presence of repair matrix. Relative values normalized to FUT8::TevI. Data (a,b,d) are shown as the mean+s.e.m. Figure 3: Harnessing the TevI domain to create a cTALEN nickase. ( a ) Optimizing target-site position within the DNA spacer. A series of asymmetric targets (schematic, top) were generated that contain a sliding CAACGC target sequence within a fixed 15-bp DNA spacer region. Relative activity is based on a yeast SSA assay ( n =3). TBS-L and TBS-R, TBS for the left and right monomers, respectively. ( b ) cTALEN nickase activity as a function of DNA spacer. A series of asymmetric targets (schematic, left) were created containing two TBS (TBS-L and TBS-R), each with a flanking TevI target site (C and C′), juxtaposed with the 3′ ends proximal (tail-to-tail) and separated by spacer DNA ranging from 8 to 24 bp between distal nicking sites. Assays ( n =3) performed as in ( a ). ( c ) Overview of the in vivo gene modification assay used for characterizing activity. The repair matrix consists of two homologous regions (LH, left homology; RH, right homology) flanking a 29 bp insert (*). Targeted cleavage stimulates DNA repair either through NHEJ or HDR with the provided matrix, resulting in alternative disruptions (xxx versus *, respectively) of the TTS region. Events are detected via amplicon sequencing using outside primers flanking the homology arms. ( d ) TevI-based TALENs promote targeted gene disruption at endogenous loci. TALENs targeting the alpha1-6-fucosyltransferase (RVD designation FUT8) gene in CHO-K1 cells were assayed ( n =3) as outlined ( c ) in the absence of a repair matrix. cFUT8L, RVD designation for left TDBS in a cTALEN context. (ε), enhancer reagent TREX2. Neg. Ctl, transfection with empty vector. ( e ) cTALEN nickases promote TGC. TGC efficacy, calculated as the ratio of HDR:NHEJ events, for assays in CHO-K1 cells as outlined ( c ) in the presence of repair matrix. Relative values normalized to FUT8::TevI. Data ( a , b , d ) are shown as the mean+s.e.m. Full size image Recent studies [43] , [44] , [45] have highlighted the need and benefit of using nickases rather than cleavases to promote targeted gene correction (TGC). Inducing homology-directed repair (HDR) via a single-strand break, although less efficient, avoids deleterious events such as mutagenic non-homologous end-joining (NHEJ) or translocations. To assess the cTALEN nickase, we adapted an endogenous gene-targeting assay that permits differential detection of mutagenic NHEJ versus HDR ( Fig. 3c ). We observed substantial gene modification activity ( Fig. 3d ) for the two standard-configuration TALENs tested (FUT8::FokI, 18%; FUT8::TevI, 3.2%), with NHEJ levels being unaffected by the presence of the repair matrix. In both cases, overall indel events were centred within the TTS as seen previously for the NPT5::FokI TALEN ( Fig. 2d ). Remarkably, although FUT8::TevI was ~6-fold less effective than FUT8::FokI, activity could essentially be rescued (FUT8::TevI(ε), 16%) by an enhancer molecule such as three-prime repair exonuclease 2 (TREX2). As DNA double-strand cleavage by the TevI CD liberates 2-nt 3′ overhangs, end processing by TREX2 can be used to drive mutagenic NHEJ before the precise rejoining of the induced breaks [46] , [47] . For all TALEN monomers, however, NHEJ activity could not be observed (only cFUT8L::TevI shown) even with added TREX2, presumably because at least one DNA strand remains intact. When the repair matrix was included, HDR events were detectable for the two standard TALENs (FUT8::FokI, 1.1%; FUT8::TevI, 0.10%) and one of the TevI-based monomers (cFUT8L::TevI, 0.11%), demonstrating that a cTALEN nickase can effect TGC at an endogenous locus. As for TevI::TALEs, no detectable TALE::TevI-related toxicity was observed in a CHO-K1 cell survival assay ( Supplementary Fig. S5 ). The relative TGC efficacy (>25-fold compared with the FokI-based TALEN), calculated as a ratio of NHEJ to HDR, further highlights the utility and safety of nickases for minimizing deleterious gene modification events ( Fig. 3e ). Site-specific genome engineering using designer nucleases (for example, LHEs, ZFNs or TALENs) is a preeminent biotechnology with a diverse range of downstream applications [1] , [3] . With the promise of readily available (that is, 4–6 weeks), highly-specific (that is, non-toxic) targeted nucleases [24] , [25] , [36] , [37] , [38] , TALENs are quickly becoming the de facto standard, surpassing the ubiquitous ZFN technology. Still, today’s TALEN technology necessitates introducing three to four times as much material for equivalent ZFN constructs, a cost that is currently borne as ZFNs in many cases are perceived sub-par to TALENs for specificity [26] . The immediate importance of further developing TALE-based nucleases is thus twofold. Scientifically, access to a single-chain, reduced-size and highly targetable nuclease is invaluable. Delivery of large DNA/RNA sequences (especially in primary cells, though other cell-type variations exist) can be limiting for research. Economically, generating this material (for example, transfection quality RNA) is expensive. Furthermore, for applications that use viral packaging for delivery, the material is not only highly expensive but experiments may also be unfeasible owing to size limitations in the viral payload. In this work, we drew upon the emerging TALE-based technology to develop new site-specific tools for directed genome engineering. Our cTALEN design couples a partially selective CD with the robust and programmable DNA-targeting specificity of a TALE to create single-chain nucleases ( Fig. 1b ). In a recent parallel study [15] , the CD of I-TevI was fused to a ZFP array as well as an inactivated monomeric LHE (I-OnuI) and shown to retain nuclease activity in vitro and in bacterial and yeast-based assays. We demonstrate that the partially selective TevI CD permits the creation of novel, high-fidelity TALE-based designer nucleases having significant in vivo activity in yeast, plant and mammalian systems. Notably, we show that fusion context ( Fig. 4 ) can be used to modulate the I-TevI cleavage mechanism for high-efficiency cleaving (N-terminal fusions) or nicking (C-terminal fusions). Thus, investigators interested in optimizing precise gene modification via recombination ( Fig. 3e ) can chose the C-terminal fusion architecture, while aleatory gene knockouts ( Fig. 2b ) can be achieved by the N-terminal fusion architecture. 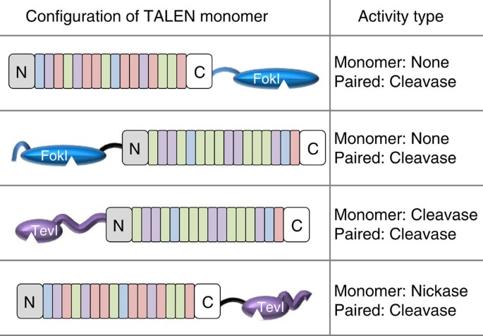Figure 4: Schematic of TALE monomer configurations. Monomer, activity when only a single TBS is present in the target site. Paired, activity when two TBSs are appropriately partnered (N–/N–, N–/C– or C–/C– terminally) to allow for detection of activity. Figure 4: Schematic of TALE monomer configurations. Monomer, activity when only a single TBS is present in the target site. Paired, activity when two TBSs are appropriately partnered (N–/N–, N–/C– or C–/C– terminally) to allow for detection of activity. Full size image cTALENs offer greater flexibility via a reduced vectorization payload while maintaining the significant in vivo gene-targeting activity associated with current TALEN designs. Importantly, existing high-throughput TALE synthesis platforms can be easily adapted to use the new architecture by simply changing the RVD destination scaffold. TevI-derived cTALENs, with a sequence space limited in practice to one effective site every ~64 bases, represent the first line in the next generation of TALE-based nucleases. The cTALEN architecture additionally provides a foundation for exploring the influence of the linkage between functionally independent domains. For example, our ongoing efforts to further reduce the cTALEN size have yielded an alternative design, TevI 137 ::TALE ( Supplementary Fig. S6 ), that enhances the robustness of the original cTALEN ( Supplementary Table S1 and Supplementary Fig. S7 ). Such optimization strategies provide insight towards developing functional cohesion between fusion partners, perhaps adding an additional layer of control to reduce unwanted off-site targeting. By applying other partially selective domains, for example, low-affinity reengineered variants of LHEs, this concept should be extendable to construct a library of targetable nuclease scaffolds whose absolute specificity, driven by the TALE moiety, is suitable for therapeutic applications ( Table 1 ). Construct assembly To generate the cTALEN scaffold, DNA coding for the CD (residues 1–183) of I-TevI was amplified by the PCR using primers to introduce either N- ( Bam HI) or C-terminal ( Kpn 2I) restriction sites. Standard molecular biology techniques were used to individually fuse these sequences to DNA coding for a truncated (ΔN152/ΔC220) AvrBs3-derived TALE scaffold lacking the central repeat region. RVD ‘arrays’ containing the repeat regions (16–18 repeats total) that target given DNA sequences were subsequently cloned into these base scaffolds to create the final cTALENs ( Supplementary Fig. S6 ). To distinguish the configuration of the CD fusions, construct names are written as either CD::TALE–RVD (CD is fused N-terminal to the TALE domain) or TALE–RVD::CD (CD is fused C-terminal to the TALE domain), where TALE–RVD designates the sequence recognized by the TALE domain and CD is the CD type. Complete cTALEN scaffolds were finally cloned into vectors pCLS17403, pCLS17692 or pCLS17693 for expression in yeast, mammalian or plants, respectively. Standard TALEN constructs used as controls were synthesized by Cellectis. Target clones for single-strand annealing assays DNA targets used in the yeast screening and mammalian SSA assays were inserted into LacZ reporter vectors (pFL39-ADH-LACURAZ for yeast and pcDNA3.1-LAACZ for mammalian cells; previously described in Arnould et al . [12] ) using the Gateway protocol (Invitrogen). Yeast reporter vectors were used to transform Saccharomyces cerevisiae strain FYBL2-7B ( MAT a, ura3D851, trp1D63, leu2D1 and lys2D202 ). Targets for the plant SSA assay were inserted into YFP reporter vector pCLS14145 using standard molecular biology techniques. All targets contain a control I-SceI target site to monitor baseline SSA activity. A general overview of the SSA assay is illustrated in Supplementary Fig. S8 . Mating of TALEN-expressing clones and screening in yeast A colony gridder (QpixII, Genetix) was used for the mating of yeast strains. Mutants were gridded on nylon filters placed on YPGlycerol plates, using high gridding density (about 20 spots per cm 2 ). A second gridding process was performed on the same filters for spotting of a second layer consisting of reporter-harbouring yeast strains for each target. Membranes were placed on solid agar containing YPGlycerol-rich medium and incubated overnight at 30 °C to allow mating. Filters were then transferred onto synthetic medium, lacking leucine and tryptophan, with glucose (2%) as the carbon source (and with G418 for co-expression experiments), and incubated for 5 days at 30 °C to select for diploids carrying the expression and target vectors. Finally, filters were transferred onto YPGalactose-rich medium for 2 days at either 30 °C (stringent) or 37 °C (standard) to induce the expression of the TALEN. Filters were then placed on solid agarose medium with 0.02% X-Gal in 0.5 M sodium phosphate buffer, pH 7.0, 0.1% SDS, 6% dimethyl formamide, 7 mM β-mercaptoethanol, 1% agarose and incubated at 37 °C to monitor β-galactosidase activity. Filters were scanned and each spot was quantified using the median values of the pixels constituting the spot. We attribute the arbitrary values 0 and 1 to white and dark pixels, respectively. β-Galactosidase activity is directly associated with the efficiency of homologous recombination. Relative values are determined with respect to a positive control known to saturate the signal under the conditions tested. Extrachromosomal assay in CHO-K1 cells CHO-K1 cells were transfected with TALEN expression vectors and the reporter plasmid using Polyfect transfection reagent in accordance with the manufacturer’s protocol (Qiagen). Culture medium was removed 72 h post transfection and lysis/detection buffer was added for the β-galactosidase liquid assay. One litre of lysis/detection buffer contains: 100 ml of lysis buffer (10 mM Tris-HCl pH 7.5, 150 mM NaCl, 0.1% Triton X-100, 0.1 mg ml −1 bovine serum albumin, protease inhibitors), 10 ml of 100 × Mg buffer (100 mM MgCl 2 , 35% 2-mercaptoethanol), 110 ml of an 8 mg ml −1 solution of ONPG and 780 ml of 0.1 M sodium phosphate pH 7.5. The OD 420 is measured after incubation at 37 °C for 2 h. The entire process was performed using a 96-well plate format on an automated Velocity11 BioCel platform (BioCel). Conditions have been adapted so that the cell number and transfection efficiency are constant in all wells within the plates. To ensure experimental reproducibility, control wells are included in all plates and correlation between intra- and interplate controls allows for assay validation. Extrachromosomal assay in tobacco plant protoplasts Tobacco protoplasts were isolated and transformed using adapted methods of protocols previously described [48] . To account for the differences in the size of the various TALEN architectures, different amounts of each plasmid were used to ensure equimolar concentration in the transformations. SSA reporter plasmids (20 μg) were co-transformed with 3 pmol nuclease plasmids in protoplast SSA assays or gene-targeting experiments. YFP-positive cells were quantified by flow cytometry using a FACSCanto II (Becton, Dickinson and Company) equipped with a 488-nm solid sapphire 20 mW laser for excitation. YFP fluorescence was detected with an FITC 530/30-nm band-pass filter, and red spectrum auto-fluorescence (RSA) from living protoplasts (due to chlorophyll) was detected with a 670-nm long-pass filter in the PcrCP channel. The forward scatter and side light scatter detectors were set to 130 and 250 V, respectively. For each sample, 2 × 10 4 protoplasts were analysed and gated according to YFP and RSA values. The gate boundaries were defined using negative controls (protoplasts that were transformed with a target plasmid alone). Data were analysed by FlowJo (Tree Star Inc., OR). Cell survival assay The CHO-K1 cell line was used to seed a 96-well plate at a density of 2 × 10 5 cells per well. The next day, varying amounts of TALEN expression vectors and a constant amount of green fluorescent protein (GFP)-encoding plasmids were used to transfect the cells using Polyfect transfection reagent in accordance with the manufacturer’s protocol (Qiagen). GFP levels were monitored by flow cytometry (Guava EasyCyte, Guava Technologies) on days 1 and 6 post transfection. Cell survival is expressed as a percentage and was calculated as a ratio: TALEN-transfected cells expressing GFP on day 6/control transfected cells expressing GFP on day 6, corrected for the transfection efficiency determined on day 1. Monitoring targeted mutagenesis CHO-K1 cells (1 × 10 6 cells) were electroporated with the Nucleofector Kit T for CHO-K1 cells (Lonza) according to the manufacturer’s protocol. Cells were transfected with 5 μg of cTALEN-expressing vector or 5 μg of each TALE half for standard heterodimeric TALENs, then plated in a 10 cm dish in complete medium (F-12K medium (Gibko) supplemented with 2 mM L -glutamine, penicillin (100 IU ml −1 ), streptomycin (100 μg ml −1 ), Fungizone (0.25 μg ml −1 ) and 10% fetal bovine serum). Three days post transfection, genomic DNA was extracted (DNeasy Blood and Tissue Kit, Qiagen) and the sequence of interest amplified with specific primers flanking the endogenous target site (300–500 bp final product size). Amplicon sequencing was performed using a 454 system (454 Life Sciences), with an average of 5,000 sequence reads per sample analysed. NHEJ events were considered if insertions or deletions were detected within 2 bp of the expected cleavage site. Monitoring TGC A sequence was chosen from the alpha1-6-fucosyltransferase ( fut8 ) gene in CHO-K1 cells that contains a centralized TevI target site, and standard heterodimeric FokI- and TevI-based TALENs were synthesized. A 210-bp linear donor matrix was constructed using two oligonucleotides containing left and right homology arms of 100 and 70 bp, respectively, to the targeted region of the fut8 locus. An exogenous DNA fragment of 29 bp (5′-ttaaggcgcgccggaccgcggccgcaatt-3′) was inserted between the arms to simultaneously disrupt the TevI cleavage site and TBS spacing, thereby inhibiting further nuclease action at targeted sites. Experiments were performed by transfecting CHO-K1 cells as described above with the respective TALEN plasmids, as either heterodimers (5 μg each, 10 μg total) or monomers (5 μg total) in the absence or presence of the matrix (2 μg), followed by event detection via amplicon sequencing of genomic DNA (454 Life Sciences). This setup enabled simultaneous detection of both targeted integration of the 29-bp exogenous fragment and induced targeted mutagenesis events. How to cite this article: Beurdeley, M. et al . Compact designer TALENs for efficient genome engineering. Nat. Commun. 4:1762 doi: 10.1038/ncomms2782 (2013).